Hydrophobic handoff for direct delivery of peroxisome tail-anchored proteins Tail-anchored (TA) proteins are inserted into membranes post-translationally through a C-terminal transmembrane domain (TMD). The PEX19 protein binds peroxisome TA proteins in the cytoplasm and delivers them to the membrane through the PEX3 receptor protein. An amphipathic segment in PEX19 promotes docking on PEX3. However, how this leads to substrate insertion is unknown. Here we reconstitute peroxisome TA protein biogenesis into two sequential steps of substrate TMD engagement and membrane insertion. We identify a series of previously uncharacterized amphipathic segments in PEX19 and identify one whose hydrophobicity is required for membrane insertion, but not TMD chaperone activity or PEX3 binding. A membrane-proximal hydrophobic surface of PEX3 promotes an unconventional form of membrane intercalation, and is also required for TMD insertion. Together, these data support a mechanism in which hydrophobic moieties in the TMD chaperone and its membrane-associated receptor act in a concerted manner to prompt TMD release and membrane insertion. A fundamental problem faced by eukaryotic cells is how to target membrane proteins from cytoplasmic ribosomes to the lipid bilayer of the appropriate intracellular organelle. This problem is particularly acute for tail-anchored (TA) proteins, which possess a single C-terminal transmembrane domain (TMD) [1] , [2] . These TMDs emerge from free cytoplasmic ribosomes after translation has terminated, and must therefore be targeted to the membrane post-translationally. TA proteins are associated with all intracellular organelles and play essential roles in diverse processes such as vesicular transport [3] , apoptosis [2] , [4] and peroxisomal matrix protein import [5] , [6] . TA proteins are targeted to their compartment of residence by distinct mechanisms (reviewed in refs 7 , 8 , 9 ). The TMD of some mitochondrial outer membrane [10] , [11] and endoplasmic reticulum (ER) TA proteins [12] can be inserted into membranes without the assistance of accessory proteins. By contrast, the majority of ER TA proteins require the Get pathway (guided entry of TA proteins) to prevent their aggregation and promote organelle-specific targeting [13] , [14] , [15] . Here, the cytoplasmic TMD recognition complex (TRC) channels ER-destined TA proteins from the ribosome to the dimeric TRC40 (Get3) ATPase [13] , [16] , [17] . Get3 cycles between open and closed conformations that depend on bound nucleotide; the open conformation is nucleotide and substrate free, whereas the closed ATP bound conformation forms a hydrophobic groove associated with substrate TMD binding [18] , [19] , [20] . ATP hydrolysis appears to precede membrane association and primes Get3 for substrate delivery [21] . This requires the ER receptor proteins Get2, which promotes initial tethering [22] , [23] , and Get1, which disrupts the closed conformation [22] , [23] , suggesting that it acts subsequently to promote substrate release. A final step in the insertion process requires Get1/Get2 TMDs, which act as membrane embedded binding sites that capture the substrate TMD, and thereby facilitate its release from Get3 (ref. 24 ). Peroxisome TA proteins can also be inserted into the membrane directly from the cytoplasm and this pathway bears some similarity to the Get pathway (reviewed in refs 25 , 26 , 27 , 28 ). Here, PEX19 recognizes nascent TA proteins as well as other peroxisome membrane proteins (PMPs) in the cytoplasm and delivers them to the peroxisome membrane by binding the PEX3 receptor. This interaction occurs through an amino-terminal segment of PEX19 (refs 29 , 30 , 31 ), which forms an amphipathic helix that intercalates a groove at the membrane distal end of PEX3 (refs 32 , 33 ). PEX3 also has a conserved membrane-proximal hydrophobic surface [32] , and mutations in this region produce defects in peroxisome maturation [34] . How this region acts to promote PEX3 function remains unclear. PEX19 recognizes PMPs [30] , [35] , [36] , [37] , [38] including the TA protein PEX26 (Pex15 in yeast) through PEX19-binding sites (membrane peroxisome targeting signals (mPTSs)), which consist of a cluster of basic and hydrophobic residues that typically flank the TMD [39] , [40] , [41] , [42] . This activity requires a globular PEX19 carboxy-terminal domain (PEX19 CTD) [30] , [38] that is sufficient to bind immobilized mPTS-bearing peptides [43] . Whether this domain is also sufficient to chaperone the TA protein TMD in the context of protein translation, or requires additional accessory factors has not been determined. Removal of mPTS sequences from the TA proteins PEX26 or FIS1 impairs their peroxisome targeting, as does PEX19 knockdown [42] , [44] . Direct targeting is further corroborated by a mammalian cell-free reaction: A complex containing PEX19 and PEX26 accumulates in a pex3 mutant cell line, and PEX26 from this complex can be targeted to peroxisomes in semi-permeabilized cells in a PEX3-dependent, but TRC40 (Get3)-independent, manner [45] . A ternary complex between PEX19, PEX26 and PEX3 has also been detected [46] . However, unlike Get3 (TRC40), where a basic mechanism for TMD binding and release is known [8] , [22] , these aspects of PEX19 function remain unclear. By contrast to direct targeting in mammalian cells, studies in budding yeast suggest that the PEX26 orthologue, Pex15, is a Get3 substrate and traffics to peroxisomes through the ER [14] , [47] . In this case, PEX19 is implicated as a sorting receptor for the production of pre-peroxisomal vesicles and is proposed to execute this function through the combined action of Pex3 and mPTS binding [28] , [48] , [49] . Direct and indirect pathways for TA protein biogenesis are not mutually exclusive. However, whether these represent conserved alternate pathways or are fixed in a species-dependent manner remains unclear, and this warrants the investigation of PEX19 function in additional taxa. Also, a mechanistic understanding of how PEX19 functions is still lacking, and will help to resolve its action in these disparate capacities. Here we develop a cell-free targeting assay that employs model TA proteins and chaperones from the multicellular fungus Neurospora crassa . We find that PEX19 but not GET3 can prevent the aggregation of nascent PEX26 and promote its insertion into the peroxisome bilayer. These data support a direct targeting pathway that is conserved between mammals and filamentous fungi. Chaperone activity depends on hydrophobic contacts and requires an amphipathic segment in the CTD. We identify an additional PEX19 amphipathic segment that lies between the PEX3-binding segment and CTD. Hydrophobicity in this area is required for TMD insertion but not chaperone activity or PEX3 binding. The hydrophobic surface at the base of PEX3 promotes an unconventional form of membrane association, and is also required for TMD insertion. Together, these data support a model in which hydrophobic moieties in PEX19 and PEX3 act in distinct capacities to promote TMD release and insertion. A cell-free assay for PEX19 and GET3 chaperone activities We initiated this study by constructing model TA proteins consisting of enhanced green fluorescent protein (GFP)-fused TMDs and flanking sequences from peroxisome ( Neurospora PEX26: TMD-PEX26), and ER-resident ( Neurospora SEC61β: TMD-SEC61β) TA proteins ( Supplementary Fig. 1 ). To assess targeting in the cell, mRNA was prepared from these constructs and microinjected into animal cells (normal rat kidney cells) along with markers of the ER or peroxisome matrix. After several hours of incubation, newly synthesized TMD-PEX26 is exclusively peroxisome associated, while TMD-SEC61β is localized to the ER ( Fig. 1a ). Thus, these model TA proteins possess all the necessary information for organelle-specific targeting. 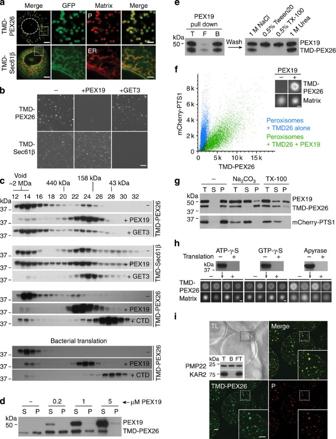Figure 1: Reconstitution of peroxisome TA protein biogenesis. (a) mRNAs encoding model peroxisome (TMD-PEX26) or ER (TMD-SEC61β) TA proteins were microinjected along with markers of peroxisome matrix (P=mCherry-PTS1) or ER lumen (ER=mCherry-KDEL). After several hours, localization of mRNA translation products was assessed by confocal microscopy. The left panels show an overview of the cell. Scale bar, 8 μm. The dotted circle shows the position of the nucleus and the dotted box indicates the region that is magnified in the three right panels. Scale bar, 2 μm. (b) The indicated GFP-TMD mRNAs were translated in the absence and presence of recombinant PEX19 or GET3. Aggregates were visualized by fluorescence microscopy. Scale bar, 2 μm. (c) The indicated translation reactions were analysed by gel filtration. Fractions along with void volume and size markers are indicated. Translation reactions utilizing a bacterial translation system are labelled bacterial translation. The PEX19 C-terminal domain is referred to as CTD. (d) TMD-PEX26 was translated in the presence of varying amounts of PEX19 and the reaction was centrifuged at 100kgto produce pellet (P) and supernatant (S) fractions. Both TMD-PEX26 and PEX19 are HA tagged. This figure is complemented bySupplementary Figs 2 and 5. (e) Detergent treatment releases TMD-PEX26 from PEX19. TMD-PEX26/PEX19 complexes were pulled down with a His-tag on PEX19, and then washed with the indicated conditions followed by anti-HA western blotting. (f) PEX19 delivers TMD-PEX26 to the peroxisome membrane. Flow cytometry shows that the majority of mCherry-labelled peroxisomes receive TMD-PEX26. The inset panels show typical rings of peroxisome-associated TMD-PEX26. Scale bar, 1 μm. This figure is complemented bySupplementary Figs 3 and 5. (g) Peroxisome-associated TMD-PEX26 is resistant to extraction by sodium carbonate. Membranes from the cell-free reaction were extracted with the indicated treatments. Total (T), supernatant (S) and pellet (P) fractions are analysed. The lower panel shows behaviour of the matrix marker mCherry-PTS1. (h) The effect of apyrase and the indicated nonhydrolyzable nucleotide analogues on TMD-PEX26 translation (upper panels) and targeting (lower panels). Scale bar, 1 μm. This figure is complemented bySupplementary Fig. 4. (i) ER membranes are not required for cell-free targeting. Peroxisomes were immunoisolated, and total (T), bead (B) and flow-through (FT) fractions were analysed by western blotting for PMP22-HA and the ER marker, KAR2 (inset panel). Isolated peroxisomes (on sepharose beads) were incubated with PEX19/TMD-PEX26 complexes and then examined by confocal microscopy for the localization of TMD-PEX26 and peroxisomes (P). Scale bar, 2 μm. Sepharose beads are seen in the TL panel. The dotted box indicates the region that is magnified in the inset panels. Scale bar, 1 μm. TL, transmitted light microscopy. Figure 1: Reconstitution of peroxisome TA protein biogenesis. ( a ) mRNAs encoding model peroxisome (TMD-PEX26) or ER (TMD-SEC61β) TA proteins were microinjected along with markers of peroxisome matrix (P=mCherry-PTS1) or ER lumen (ER=mCherry-KDEL). After several hours, localization of mRNA translation products was assessed by confocal microscopy. The left panels show an overview of the cell. Scale bar, 8 μm. The dotted circle shows the position of the nucleus and the dotted box indicates the region that is magnified in the three right panels. Scale bar, 2 μm. ( b ) The indicated GFP-TMD mRNAs were translated in the absence and presence of recombinant PEX19 or GET3. Aggregates were visualized by fluorescence microscopy. Scale bar, 2 μm. ( c ) The indicated translation reactions were analysed by gel filtration. Fractions along with void volume and size markers are indicated. Translation reactions utilizing a bacterial translation system are labelled bacterial translation. The PEX19 C-terminal domain is referred to as CTD. ( d ) TMD-PEX26 was translated in the presence of varying amounts of PEX19 and the reaction was centrifuged at 100k g to produce pellet (P) and supernatant (S) fractions. Both TMD-PEX26 and PEX19 are HA tagged. This figure is complemented by Supplementary Figs 2 and 5 . ( e ) Detergent treatment releases TMD-PEX26 from PEX19. TMD-PEX26/PEX19 complexes were pulled down with a His-tag on PEX19, and then washed with the indicated conditions followed by anti-HA western blotting. ( f ) PEX19 delivers TMD-PEX26 to the peroxisome membrane. Flow cytometry shows that the majority of mCherry-labelled peroxisomes receive TMD-PEX26. The inset panels show typical rings of peroxisome-associated TMD-PEX26. Scale bar, 1 μm. This figure is complemented by Supplementary Figs 3 and 5 . ( g ) Peroxisome-associated TMD-PEX26 is resistant to extraction by sodium carbonate. Membranes from the cell-free reaction were extracted with the indicated treatments. Total (T), supernatant (S) and pellet (P) fractions are analysed. The lower panel shows behaviour of the matrix marker mCherry-PTS1. ( h ) The effect of apyrase and the indicated nonhydrolyzable nucleotide analogues on TMD-PEX26 translation (upper panels) and targeting (lower panels). Scale bar, 1 μm. This figure is complemented by Supplementary Fig. 4 . ( i ) ER membranes are not required for cell-free targeting. Peroxisomes were immunoisolated, and total (T), bead (B) and flow-through (FT) fractions were analysed by western blotting for PMP22-HA and the ER marker, KAR2 (inset panel). Isolated peroxisomes (on sepharose beads) were incubated with PEX19/TMD-PEX26 complexes and then examined by confocal microscopy for the localization of TMD-PEX26 and peroxisomes (P). Scale bar, 2 μm. Sepharose beads are seen in the TL panel. The dotted box indicates the region that is magnified in the inset panels. Scale bar, 1 μm. TL, transmitted light microscopy. Full size image We next translated these mRNAs in a HeLa cell translation extract (see Methods) in the presence and absence of recombinant Neurospora PEX19 or GET3. The fate of TA proteins was followed using fluorescence microscopy, gel filtration and ultracentrifugation. By themselves, both TMD-PEX26 and TMD-SEC61β form large aggregates seen as punctate structures by fluorescence microscopy ( Fig. 1b ). Aggregates are further observed based on elution in the void volume during gel filtration ( Fig. 1c ). Translation in the presence of PEX19 prevents aggregation of TMD-PEX26, but has no effect on TMD-SEC61β. By contrast, GET3 prevents aggregation of TMD-SEC61β, but not TMD-PEX26. In both cases, when translated in the presence of their cognate chaperones, TA proteins no longer form punctate structures ( Fig. 1b ), and are included in the gel filtration medium ( Fig. 1c ). The human PEX19 C-terminal domain (amino acids 161–283) is capable of binding immobilized mPTS sequences [43] . We produced the analogous fragment of Neurospora PEX19 (CTD: amino acids 208–327) and found that this domain is also sufficient for chaperone activity ( Fig. 1c ). PEX19 and the CTD also function effectively when TMD-PEX26 is produced in a bacterial translation extract, indicating that substrate engagement by PEX19 does not require additional eukaryotic factors ( Fig. 1c , bacterial translation). The chaperone activity of PEX19 was further assessed by ultracentrifugation. TMD-PEX26 aggregates are found in the pellet following ultracentrifugation, and increasing amounts of PEX19 render TMD-PEX26 increasingly soluble ( Fig. 1d ). Here, both PEX19 and TMD-PEX26 are tagged N-terminally with the human influenza haemaglutinin (HA) epitope and their similar recognition by western blotting ( Supplementary Fig. 2 ) allows an approximation of relative protein levels. TMD-PEX26 is significantly shifted to the supernatant fraction by approximately equimolar PEX19 ( Fig. 1d ) and is fully soluble in the presence of fivefold excess PEX19. Thus, vast excesses of PEX19 are not required for its chaperone activity. Finally, PEX19/TMD-PEX26 complexes were immobilized on beads through a tag on PEX19, and then washed with various chemical treatments. Binding of PEX19 to TMD-PEX26 is disrupted by detergents, but resistant to 1 M NaCl or 1 M urea ( Fig. 1e ). Therefore, as with TRC40 (GET3) and its substrates [13] , hydrophobic contacts mediate the association between PEX19 and TMD-PEX26. TMD-PEX26 insertion does not require ATP hydrolysis TMD-PEX26 was next translated into the HeLa extract in the presence or absence of PEX19. mCherry-PTS1-labelled Neurospora peroxisomes were then added, followed by a second incubation. Fluorescence microscopy shows that TMD-PEX26 is targeted to these peroxisomes if synthesized in the presence, but not absence, of PEX19. Flow cytometry further reveals that the entire peroxisome population shifts to a GFP-positive status, indicating that the majority of peroxisomes receive TMD-PEX26 ( Fig. 1f ). Importantly, peroxisome-associated TMD-PEX26 is fully resistant to carbonate extraction, indicating its integration into the bilayer ( Fig. 1g ). To estimate how many rounds of import are supported by the cell-free reaction, we compared levels of carbonate resistant TMD-PEX26 and the PEX19 receptor, PEX3. A standard import assay produces a TMD-PEX26-to-PEX3 ratio of around 15 ( Supplementary Fig. 3 ), suggesting that each PEX3 molecule is engaged in multiple rounds of import. We next examined the energy requirements of this reaction by depleting ATP with apyrase, or by adding nonhydrolyzable analogues of ATP (ATPγS) or GTP (GTPγS; Fig. 1h ; Supplementary Fig. 4 ). To control for the efficacy of these treatments, they were conducted before translation, in which case protein synthesis is abolished. By contrast, identical treatments made after translation, but before the addition of peroxisomes, had no effect on TMD-PEX26 targeting, suggesting that PEX19-mediated membrane insertion occurs independently of ATP and GTP hydrolysis. We also farnesylated [50] recombinant PEX19 on its C-terminal CAAX box [51] and found that this modification does not have a major impact on PEX19 function in the cell-free reaction. We further found that the CAAX box is dispensable for PEX19 function in vivo ( Supplementary Fig. 5 ). To determine the activity of PEX19 on other substrates, we fused TMD segments from Neurospora FIS1 (TMD-FIS1) and a predicted Neurospora TA protein kinase (TMD-STK36) [52] to the C terminus of GFP ( Supplementary Fig. 1 ). Microinjection of mRNA encoding these proteins into mammalian cells reveals that both are targeted to peroxisomes as well as mitochondria ( Supplementary Fig. 6 ). In the cell-free assay, PEX19 stimulates peroxisome targeting of both TMD-FIS1 and TMD-STK36. Both chaperone and targeting activities are weak compared with its action on TMD-PEX26, and this may relate to the dual localization of these particular substrates. Nevertheless, these results show that PEX19 can also act on these substrates in vitro . TMD-PEX26 insertion occurs in the absence of ER membranes Previous studies have implicated the ER in PMP biogenesis [47] . To remove ER from the cell-free reaction, peroxisomes were immunoisolated on antibody-coated sepharose beads (see Methods ). In addition, TMD-PEX26 was produced in a bacterial translation system to further exclude the influence of the TRC and other eukaryotic factors that might be present in the HeLa translation extract. Western blotting confirmed that purified peroxisomes are free of the ER-resident KAR2 protein ( Fig. 1i ). PEX19 efficiently delivers TMD-PEX26 to these peroxisomes ( Fig. 1i ), indicating that it can function in the absence of detectable ER membranes. Conversion of TMD-PEX26 to a GET3 substrate We next sought to evaluate the role of TMD hydrophobicity in TMD-PEX26 by mutating three small or charged residues to leucine to produce TMD-PEX26-3L ( Supplementary Fig. 1 ). In the cell-free system, this variant is still chaperoned by PEX19 ( Fig. 2a ), but is defective in integration to the peroxisome membrane ( Fig. 2b ; Supplementary Fig. 7 ), suggesting that insertion is sensitive to TMD hydrophobicity downstream of PEX19 engagement. GET3 can chaperone TMD-PEX26-3L ( Fig. 2a ) and its targeting to both ER and peroxisomes in vivo ( Fig. 2c ) confirms recognition by both insertion machineries. These findings imply that low overall TMD hydrophobicity normally excludes PEX26 from GET3 recognition. 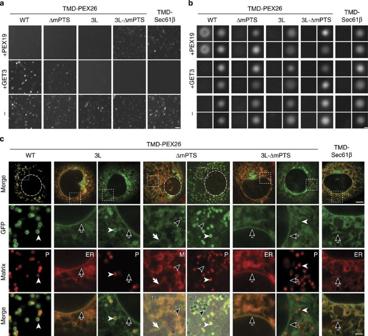Figure 2: Conversion of a peroxisome TA protein into a GET3 substrate. (a) The indicated TMD-PEX26 variants were translated in the presence or absence of the indicated recombinant chaperones and GFP was imaged using fluorescence microscopy. Scale bar, 2 μm. (b) Peroxisome targeting of the same TMD-PEX26 variants and chaperone combinations shown ina. Scale bar, 1 μm. This figure is complemented bySupplementary Fig. 7. (c) mRNA encoding the indicated GFP-TMD fusion proteins was microinjected into natural rat kidney cells, which were imaged after several hours of incubation. The upper row shows an overview of the indicated cells. The dotted circles show the position of the nucleus. The dotted box indicates the region that is magnified in the three lower panels in each column. Scale bar, 2 μm. ER (black arrows) was identified by injection of mRNA encoding a mCherry-KDEL fusion protein. Peroxisomes (P, white arrowhead) were labelled by co-injection of purified recombinant mCherry-PTS1. Mitochondria (M, white arrow) were labelled with mitotracker and putative lipid droplets (black arrowhead) were identified by transmitted light microscopy (+TL). Figure 2: Conversion of a peroxisome TA protein into a GET3 substrate. ( a ) The indicated TMD-PEX26 variants were translated in the presence or absence of the indicated recombinant chaperones and GFP was imaged using fluorescence microscopy. Scale bar, 2 μm. ( b ) Peroxisome targeting of the same TMD-PEX26 variants and chaperone combinations shown in a . Scale bar, 1 μm. This figure is complemented by Supplementary Fig. 7 . ( c ) mRNA encoding the indicated GFP-TMD fusion proteins was microinjected into natural rat kidney cells, which were imaged after several hours of incubation. The upper row shows an overview of the indicated cells. The dotted circles show the position of the nucleus. The dotted box indicates the region that is magnified in the three lower panels in each column. Scale bar, 2 μm. ER (black arrows) was identified by injection of mRNA encoding a mCherry-KDEL fusion protein. Peroxisomes (P, white arrowhead) were labelled by co-injection of purified recombinant mCherry-PTS1. Mitochondria (M, white arrow) were labelled with mitotracker and putative lipid droplets (black arrowhead) were identified by transmitted light microscopy (+TL). Full size image Two mPTS sequences are found in PEX26; one directly flanking the TMD and the other at the extreme C terminus [42] . We deleted the C-terminal mPTS to produce TMD-PEX26-ΔmPTS. This variant is still chaperoned by PEX19 ( Fig. 2a ). However, its cell-free peroxisome targeting is partially impaired ( Fig. 2b ; Supplementary Fig. 7 ). Defects in trafficking are further seen in vivo , where TMD-PEX26-ΔmPTS localizes to mitochondria and putative lipid droplets in addition to peroxisomes ( Fig. 2c ). The partial defects observed on the deletion of one mPTS in TMD-PEX26 are largely consistent with findings obtained with mammalian PEX26 where deletion of both mPTS sequences is required to fully abolish PEX19 recognition and peroxisome targeting in vivo [45] . Finally, these two changes were combined to create TMD-PEX26-3L-ΔmPTS. This variant is no longer chaperoned by PEX19 ( Fig. 2a ) nor integrated to the peroxisome membrane in the cell-free system ( Fig. 2b ; Supplementary Fig. 7 ). By contrast, TMD-PEX26-3L-ΔmPTS is chaperoned by GET3 and its in vivo targeting is restricted to the ER ( Fig. 2c ), indicating conversion to an exclusive GET3 substrate. Together, these data show that low overall hydrophobicity excludes TMD-PEX26 from recognition by GET3, while the mPTS promotes peroxisome targeting. Distinct functions of PEX19 amphipathic segments We next sought to determine the nature of protein–protein interactions underlying PEX19 chaperone and targeting activities. We scrutinized the region that lies between the N-terminal PEX3-binding segment and C-terminal mPTS-binding domain and identified four previously uncharacterized amphipathic segments (alpha-b, -c, -d, and -e) that are embedded within a region of intrinsic disorder ( Fig. 3a ; Supplementary Fig. 8 ) [38] . When viewed by helical wheel projections, hydrophobicity in these segments consists of four to five residues (generally, L, V, I and M), and based on their degree of hydrophobicity, these regions bear some similarity to the PEX3-docking segment, which we refer to here as alpha-a. Interestingly, a helix projecting from the globular C-terminal mPTS-binding domain of human PEX19 (alpha-1 according to ref. 43 ) also conforms to this pattern ( Fig. 3b–d ). Similar segments could also be identified in yeast and human PEX19, and of all these regions, alpha-a, -d, -e and -1 are most highly conserved ( Fig. 3c ; Supplementary Fig. 8 ). Alpha-a and alpha-d contain phenylalanine residues at the end (alpha-a) or the beginning (alpha-d) of the hydrophobic segment. This arrangement is evolutionarily conserved with the exception of Saccharomyces cerevisiae and closely related species, where the aromatic residue is at the beginning rather than the end of alpha-a ( Fig. 3c ; Supplementary Fig. 9 ). 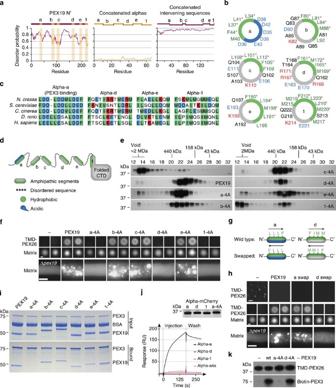Figure 3: Amphipathic segments of PEX19 play distinct roles in chaperone and targeting activities. (a) Identification of amphipathic segments in the PEX19 N-terminal domain. Theyaxis indicates the predicted probability of disorder. Amphipathic segments are labelled. Disorder probability was also calculated for concatenated amphipathic (middle panel) and intervening sequences (right panel). This figure is complemented bySupplementary Fig. 8. (b) Helical wheel projections ofNeurosporaamphipathic segment. Hydrophobic residues are coloured green, acidic residues are blue and basic residues are red. Asterisks mark the residues mutated to alanine to make the alpha 4A mutants. This figure is complemented bySupplementary Fig. 8. (c) A sequence alignment shows conservation of the indicated amphipathic segments. Colouring is according tob. This figure is complemented bySupplementary Fig. 8. (d) The schematic shows the overall structure of PEX19. Features are labelled and specified in the legend. CTD, C-terminal domain. (e) Chaperone activity of the indicating PEX19 4A mutants by gel filtration. Fractions along with void volume and size markers are indicated. This figure is complemented bySupplementary Fig. 10. (f) Function of the indicated PEX19 4A mutants in cell-free targeting (upper panels, scale bar, 1 μm) and ability to complement a pex19 deletion strain (lower panels, scale bar, 10 μm) as assessed by matrix protein (mCherry-PTS1) import. This figure is complemented bySupplementary Fig. 15a. (g) The schematic depicts hydrophobic residues of alpha-a and alpha-d and their swapped variants. This figure is complemented bySupplementary Fig. 9. (h) The indicated PEX19 variants were assayed for chaperone activity (upper panels, scale bar, 2 μm), cell-free targeting (middle panels, scale bar, 1 μm) and complementation of the pex19 deletion strain (lower panels, scale bar, 10 μm). This figure is complemented bySupplementary Fig. 15b. (i) Pull-down assay reveals the ability of the PEX19 4A mutants to physically associate with bead-associated PEX3. Input and bound fractions are shown. Proteins are visualized by staining with Coomassie Brilliant Blue. (j) Surface plasmon resonance analysis of the interaction between the indicated alpha segment-mCherry fusion proteins and immobilized PEX3. For simplicity, the binding curves at a concentration of 5 μM are shown. A full data set can be found inSupplementary Fig. 11. (k) TMD-PEX26 pulls down PEX3 in the presence of PEX19 and PEX19 d-4A but not PEX19 a-4A. TMD-PEX26 was translated in the presence of the indicated PEX19 variants and then pulled down after being presented with a biotinylated version of cytoplasmic domain of PEX3. The bound fraction was separated by SDS–PAGE and analysed by western blotting against the indicated proteins. Figure 3: Amphipathic segments of PEX19 play distinct roles in chaperone and targeting activities. ( a ) Identification of amphipathic segments in the PEX19 N-terminal domain. The y axis indicates the predicted probability of disorder. Amphipathic segments are labelled. Disorder probability was also calculated for concatenated amphipathic (middle panel) and intervening sequences (right panel). This figure is complemented by Supplementary Fig. 8 . ( b ) Helical wheel projections of Neurospora amphipathic segment. Hydrophobic residues are coloured green, acidic residues are blue and basic residues are red. Asterisks mark the residues mutated to alanine to make the alpha 4A mutants. This figure is complemented by Supplementary Fig. 8 . ( c ) A sequence alignment shows conservation of the indicated amphipathic segments. Colouring is according to b . This figure is complemented by Supplementary Fig. 8 . ( d ) The schematic shows the overall structure of PEX19. Features are labelled and specified in the legend. CTD, C-terminal domain. ( e ) Chaperone activity of the indicating PEX19 4A mutants by gel filtration. Fractions along with void volume and size markers are indicated. This figure is complemented by Supplementary Fig. 10 . ( f ) Function of the indicated PEX19 4A mutants in cell-free targeting (upper panels, scale bar, 1 μm) and ability to complement a pex19 deletion strain (lower panels, scale bar, 10 μm) as assessed by matrix protein (mCherry-PTS1) import. This figure is complemented by Supplementary Fig. 15a . ( g ) The schematic depicts hydrophobic residues of alpha-a and alpha-d and their swapped variants. This figure is complemented by Supplementary Fig. 9 . ( h ) The indicated PEX19 variants were assayed for chaperone activity (upper panels, scale bar, 2 μm), cell-free targeting (middle panels, scale bar, 1 μm) and complementation of the pex19 deletion strain (lower panels, scale bar, 10 μm). This figure is complemented by Supplementary Fig. 15b . ( i ) Pull-down assay reveals the ability of the PEX19 4A mutants to physically associate with bead-associated PEX3. Input and bound fractions are shown. Proteins are visualized by staining with Coomassie Brilliant Blue. ( j ) Surface plasmon resonance analysis of the interaction between the indicated alpha segment-mCherry fusion proteins and immobilized PEX3. For simplicity, the binding curves at a concentration of 5 μM are shown. A full data set can be found in Supplementary Fig. 11 . ( k ) TMD-PEX26 pulls down PEX3 in the presence of PEX19 and PEX19 d-4A but not PEX19 a-4A. TMD-PEX26 was translated in the presence of the indicated PEX19 variants and then pulled down after being presented with a biotinylated version of cytoplasmic domain of PEX3. The bound fraction was separated by SDS–PAGE and analysed by western blotting against the indicated proteins. Full size image To determine the function of PEX19 amphipathic segments, we systematically replaced four hydrophobic residues with alanine (4A mutants) and assayed these variants in the cell-free targeting assay and for their ability to complement a Neurospora pex19 deletion strain. Chaperone activity of the alpha-1 4A mutant is significantly diminished, while all the other alpha mutants retain this capacity ( Fig. 3e ). Cell-free targeting to peroxisomes is abolished by 4A mutations in alpha-a, -d and -1 ( Fig. 3f ), and the importance of these three segments is further corroborated by their inability to support peroxisome biogenesis when present as the sole source of PEX19 function in vivo ( Fig. 3f ). Alpha-a and alpha-1 were previously associated with PEX3 binding [32] , [33] and mPTS recognition [43] , respectively. Our data identify a new functional segment in the form of alpha-d and suggest that it is not required for chaperone activity. To further exclude a role for alpha-d in this aspect of PEX19 function, we quantified the appearance of TMD-PEX26 aggregates in chaperone assays conducted with suboptimal concentrations of PEX19 ( Supplementary fig. 10 ). PEX19 and PEX19 d-4A have overlapping dose-dependent activity profiles, suggesting that their chaperone activities are identical or nearly identical. Together, these data define key roles for alpha-1 in the chaperone activity and for alpha-a and alpha-d in membrane insertion. To determine the importance of the position of conserved aromatic residues in alpha-a and -d, we constructed mutants that swap residues at the beginning and end of these segments (swapped mutants). PEX19 tolerates this change in alpha-a, with no visible impact on function in vitro and in vivo . By contrast, swapping in alpha-d abolishes cell-free targeting and severely diminishes function in vivo ( Fig. 3g,h ). The similar character of alpha segments prompted us to next examine their influence on PEX3 binding. PEX3 was immobilized on beads and pull-down assays were conducted with purified PEX19 4A mutants. As previously reported [32] , [33] , mutation of hydrophobic residues in the PEX3-docking domain (alpha-a) abolishes interaction with PEX3 ( Fig. 3i ). By contrast, all of the other alpha 4A mutants bind to PEX3 at levels comparable to wild-type PEX19. Because alpha segments may not be exposed in the full-length protein, or become exposed only at certain stages of a targeting cycle, we also determined the ability of alpha-a, -d and -1 to individually bind PEX3. Alpha segments were fused to the N terminus of mCherry and their binding to immobilized PEX3 was assessed by surface plasmon resonance (SPR). In this assay, alpha-a-mCherry interacts with PEX3, and this binding is abolished by the 4A mutation. By contrast, alpha-d and alpha-1 do not show an appreciable interaction with PEX3 ( Fig. 3j ; Supplementary Fig. 11 ). Data presented thus far suggest that alpha-d is not involved in PEX3 binding. However, such a role could be conditional and depend on the presence of bound substrate. To investigate this possibility, we translated TMD-PEX26 in the presence of PEX19 variants, added the cytoplasmic domain of PEX3 and pulled down the resulting complex with a tag on TMD-PEX26 ( Fig. 3k ). TMD-PEX26 pulls down PEX3 in the presence of PEX19 and PEX19 d-4A, but not PEX19 a-4A. Thus, alpha-d does not appear to be required for PEX3 binding. Taken together with the finding that alpha-d is dispensable for chaperone activity ( Fig. 3e ; Supplementary fig. 10 ), these data suggest that alpha-d exerts its essential function after formation of the ternary complex. PEX3 hydrophobicity required for cell-free targeting We next sought to determine the role of the membrane-proximal hydrophobic surface of PEX3 (ref. 32 ) by incorporating mutants that alter its hydrophobicity into the cell-free assay ( Fig. 4 ). Introduction of a charged (L261D) or polar (L261N) side chain in this region abolishes and severely impairs PEX3 function, respectively. A double mutant that conserves but diminishes hydrophobicity (L261A, L209A (PEX3-2A)) can promote the production of peroxisomes, but accumulates some matrix marker in the cytoplasm ( Fig. 4b ) and has fewer peroxisomes in the steady state ( Supplementary Fig. 12 ), suggesting a partial loss of function. Peroxisomes were isolated from this mutant and assessed for their ability to accept TMD-PEX26 from PEX19. Compared with wild-type peroxisomes, significantly less TMD-PEX26 is targeted to the membrane of PEX3-2A peroxisomes ( Fig. 4c ). Immunostaining of isolated peroxisomes shows that PEX3-2A is present at levels comparable to that of wild-type PEX3 ( Fig. 4c ). In the pull-down assay, recombinant PEX3-2A interacts equally well with PEX19 and PEX19 d-4A, but not with PEX19 a-4A ( Fig. 4d ). A similar interaction profile was observed with cargo-loaded PEX19 ( Supplementary Fig. 13 ). Together, these results indicate that neither diminished expression nor defects in PEX19 binding account for PEX3-2A dysfunction in TA protein insertion. Thus, this region is likely to act after recruitment of PEX19 to the membrane. 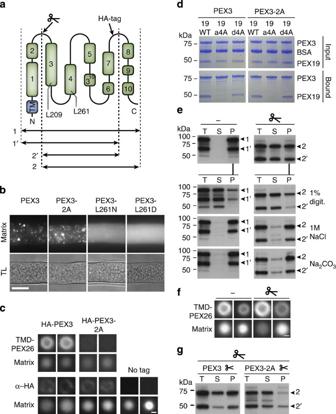Figure 4: Hydrophobicity at the base of PEX3 is required for direct TA protein targeting. (a) A schematic of PEX3 secondary structure is shown with helical segments numbered according to ref.32. Position of the TMD, HA-tag, protease site () and residues mutated to make the PEX3-2A mutant are indicated. The lower region indicates the fragments produced during treatment with PreScission protease (1, 1′, 2 and 2′). (b) Ability of the indicated PEX3 mutants to complement apex3deletion strain. Scale bar, 10 μm. Matrix is revealed by mCherry-PTS1. TL, transmitted light microscopy. This figure is complemented bySupplementary Fig. 12. (c) Mutants that disrupt the PEX3 hydrophobic surface are defective in TMD-PEX26 integration. Isolated peroxisomes from the indicated strains were used in the cell-free targeting assay and immunostained (α-HA) to assess levels of PEX3. A strain in which PEX3 is not tagged (no tag) serves as a negative control for antibody staining. Scale bar, 1 μm. (d) Pull-down assays show that PEX3-2A binds to PEX19 and PEX19 d-4A as well as wild-type PEX3. The assay was conducted as described inFig. 3i. (e) Peroxisomes derived from wild-type or PEX3 strain are incubated in the presence () and absence (−) of PreScission proteins and then fractionated by centrifugation to produce total (T), supernatant (S) and pellet (P) fractions. Pellet fractions were resuspended, extracted in the indicated solutions and then centrifuged to regenerate T, S and P fractions. Band identities are defined ina. (f) Peroxisomes in which PEX3 has been cleaved are competent for TMD-PEX26 integration. PreScission protease-treated () and -untreated (−) peroxisomes were used in the cell-free targeting assay. Scale bar, 1 μm. (g) The PEX3-2A mutant is defective in TMD-independent membrane association. Release of the PEX3 cytosolic domain by treatment with PreScission protease was assessed for the indicated versions of PEX3 as ine. Figure 4: Hydrophobicity at the base of PEX3 is required for direct TA protein targeting. ( a ) A schematic of PEX3 secondary structure is shown with helical segments numbered according to ref. 32 . Position of the TMD, HA-tag, protease site () and residues mutated to make the PEX3-2A mutant are indicated. The lower region indicates the fragments produced during treatment with PreScission protease (1, 1′, 2 and 2′). ( b ) Ability of the indicated PEX3 mutants to complement a pex3 deletion strain. Scale bar, 10 μm. Matrix is revealed by mCherry-PTS1. TL, transmitted light microscopy. This figure is complemented by Supplementary Fig. 12 . ( c ) Mutants that disrupt the PEX3 hydrophobic surface are defective in TMD-PEX26 integration. Isolated peroxisomes from the indicated strains were used in the cell-free targeting assay and immunostained (α-HA) to assess levels of PEX3. A strain in which PEX3 is not tagged (no tag) serves as a negative control for antibody staining. Scale bar, 1 μm. ( d ) Pull-down assays show that PEX3-2A binds to PEX19 and PEX19 d-4A as well as wild-type PEX3. The assay was conducted as described in Fig. 3i . ( e ) Peroxisomes derived from wild-type or PEX3 strain are incubated in the presence () and absence (−) of PreScission proteins and then fractionated by centrifugation to produce total (T), supernatant (S) and pellet (P) fractions. Pellet fractions were resuspended, extracted in the indicated solutions and then centrifuged to regenerate T, S and P fractions. Band identities are defined in a . ( f ) Peroxisomes in which PEX3 has been cleaved are competent for TMD-PEX26 integration. PreScission protease-treated () and -untreated (−) peroxisomes were used in the cell-free targeting assay. Scale bar, 1 μm. ( g ) The PEX3-2A mutant is defective in TMD-independent membrane association. Release of the PEX3 cytosolic domain by treatment with PreScission protease was assessed for the indicated versions of PEX3 as in e . Full size image To explore ways of conditionally interfering with PEX3 function, we introduced a protease cleavage site (PreScission protease) into the loop between the second and third helical segment to produce a cleavable PEX3 (PEX3; Fig. 4a ). PEX3 can fully complement a pex3 deletion strain, indicating that the cleavage site does not interfere with function. Peroxisomes from this strain were isolated and subjected to protease treatment. Uncleaved PEX3 migrates as a doublet consisting of the full-length protein and a shorter form produced by an endogenous protease activity ( Fig. 4e ). Following protease treatment, both forms shift in size consistent with nearly complete cleavage at the engineered site. Remarkably, these peroxisomes are as competent to receive TMD-PEX26 as those receiving no protease treatment ( Fig. 4f ). To investigate the basis for this surprising result, protease-treated peroxisomes were subjected to centrifugation and separated into supernatant- and peroxisome-containing pellet fractions. Approximately half of the cleaved PEX3 remains peroxisome associated after protease treatment. Sodium carbonate extraction further reveals that the majority of the cleaved protein behaves like an integral membrane protein despite no longer being covalently attached to the N-terminal TMD ( Fig. 4e ). To determine whether membrane-proximal hydrophobic residues influence this form of membrane association, we created a cleavable version of the PEX3-2A mutant (PEX3-2A) and repeated protease treatment and fractionation. Compared with PEX3, significantly more PEX3-2A is released from peroxisomes by protease treatment ( Fig. 4g ). Thus, membrane intercalation by the PEX3 cytosolic domain is associated with its TA protein insertion activity. PMPs including TA proteins are recognized by PEX19 in the cytoplasm [35] , [36] , [37] , [38] and delivered to the membrane through PEX3 (refs 29 , 30 , 31 , 32 , 33 , 45 ). However, unlike GET3, where ATP hydrolysis and conformational changes are coupled with substrate release [8] , the mechanism that prompts PEX19 to release its substrate is unknown. Here we identify a series of previously uncharacterized amphipathic segments in PEX19 ( Fig. 3 ) and show that hydrophobicity in one of these, alpha-d, is required for TA protein insertion ( Fig. 3f ), but not chaperone activity ( Fig. 3e ; Supplementary Fig. 10 ) or PEX3 binding ( Fig. 3i,k ). The PEX19 CTD was previously shown to bind isolated mPTS sequences [43] . We find that this domain is also sufficient for chaperone activity ( Fig. 1c ) and relies on hydrophobicity in an additional amphipathic segment, alpha-1, for this activity ( Fig. 3e ). Alpha-1 and alpha-d possess a similar degree of hydrophobicity, suggesting a mechanism in which alpha-d prompts substrate release by competing with alpha-1 for hydrophobic contacts with the substrate TMD ( Fig. 5 ). 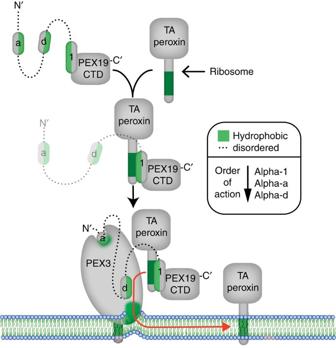Figure 5: A model for the insertion of peroxisome TA proteins. Please see the text for additional information. Figure 5: A model for the insertion of peroxisome TA proteins. Please see the text for additional information. Full size image Hydrophobicity at the base of the PEX3 is also required for TA protein insertion ( Fig. 4c ), but does not appear to play a role in PEX19 binding ( Fig. 4d ; Supplementary Fig. 13 ). This region also engenders a tight association with the bilayer ( Fig. 4e ), and therefore is likely to act downstream of PEX19 recruitment and in close proximity to the bilayer. Since this domain also binds liposomes in vitro [53] , we suggest that it functions to disrupt bilayer structure to allow the substrate TMD to breach the hydrophilic surface of the bilayer ( Fig. 5 ). Hydrophobicity in this region could also cooperate with alpha-d to prompt substrate release. Interestingly, insertion of ER TA proteins was recently shown to require membrane-embedded substrate TMD-binding sites formed by the TMDs of the Get1/Get2 receptor, which act after ATP hydrolysis and GET3 conformational changes [24] . Thus, despite their many differences, a requirement for intervention at the level of the bilayer after substrate delivery to the membrane-associated receptor may be a common feature of ER and peroxisome insertion machineries. Peroxisome TA protein insertion appears to occur in the absence of ATP hydrolysis ( Fig. 1h ) [45] and relies on the concerted action of hydrophobicity in PEX19 (alpha-d) and PEX3 (membrane-proximal hydrophobic patch). This dual requirement may act to promote compartment-specific targeting by ensuring that TMD insertion only occurs in the context of a properly configured ternary complex. Increasing the hydrophobicity of TMD-PEX26 does not abolish recognition by PEX19 ( Fig. 2a ), but insertion is defective ( Fig. 2b ) and this further supports a mechanism that depends on a finely tuned cascade of hydrophobic interactions. Alpha-a and alpha-d both have conserved aromatic residues at one end of the amphipathic segment ( Fig. 3c ). Swapping residues at the beginning and end of alpha-a does not impair its function. A similar swap occurred in a common ancestor of budding yeast and closely related species, further indicating that the position of this residue is not critical ( Supplementary Fig. 9 ). By contrast, swapping in alpha-d abrogates targeting in the cell-free assay and results in severely diminished function in vivo ( Fig. 3g,h ). Because this variant retains overall hydrophobicity, alpha-d, rather than acting as a generic hydrophobic moiety, is likely to function in a defined structural context. A side-by-side comparison shows that PEX19, but not GET3, can prevent peroxisome TA protein aggregation and promote insertion into the peroxisomal bilayer ( Fig. 1 ). Thus, as in mammalian cells [45] , Neurospora PEX26 can follow the direct PEX19-dependent pathway. TMD-PEX26 can be converted into a GET3 substrate by increasing hydrophobicity of the TMD ( Fig. 2 ). Interestingly, a similar change can also convert yeast Fis1, which is predominantly targeted to mitochondria, into a Get3 substrate [17] . Compared with GET3 substrates, PEX26 orthologues conserve a low degree of hydrophobicity ( Supplementary Fig. 14 ). Together, these observations suggest that relatively low TMD hydrophobicity is a key determinant that excludes mitochondrial and peroxisomal TA proteins from GET3 recognition. The TRC binds to Fis1 through a peripheral subunit while ER TA proteins are bound through a central subunit, suggesting that this distinction is made early in this chaperone cascade [17] . Whether peroxisome TA proteins also bind the peripheral TRC subunit and the relationship between the TRC and PEX19 await future investigation. The finding that some mitochondrial TA proteins have a predicted TMD hydrophobicity similar to that of ER TA proteins [54] undermines a simple model in which TMD hydrophobicity is a primary sorting determinant for TA proteins. In these cases, additional features of the TA protein or a more nuanced recognition of the TMD by the insertion machinery could come into play, and more work will be required to distinguish these and other possibilities. The PEX19 CTD can bind immobilized mPTS-bearing peptides [43] . This domain is also sufficient to chaperone the nascent TMD, and functions in a bacterial translation extract, indicating that TMD engagement does not require additional eukaryotic accessory factors ( Fig. 1c ). The manner in which the mPTS influences TMD binding by PEX19 remains enigmatic. Chaperone activity requires alpha-1 ( Fig. 3e ), but the extent of its hydrophobicity appears insufficient to shield a TMD from the aqueous cytoplasmic environment. We favour a model in which mPTS binding alters CTD structure to expose additional hydrophobicity to further favour TMD binding. This model can account for mPTS dependence of substrate engagement and provides a means of shielding this hydrophobicity from the cytoplasmic environment in substrate-free PEX19. Open questions also remain concerning membrane insertion of multi-pass PMPs in which each TMD does not necessarily possess an associated mPTS [40] , [41] , [55] . How these PMPs are engaged by PEX19, the extent to which they follow direct vs indirect pathways, as well as the mechanisms that determine their membrane topology are all interesting areas for future investigation. In budding yeast, TA proteins traffic through the ER [14] , [47] , [48] and Pex19 is implicated as a sorting receptor for the production of pre-peroxisomal vesicles [28] , [48] , [49] . Several of the PEX19 amphipathic segments defined here are not essential for TA protein insertion (alpha-b, -c and -e), but are relatively well conserved and could play a role in other aspects of PEX19 function. Interestingly, human PEX19 binds to PEX14 (ref. 56 ) through an FXXXF motif [57] found in the vicinity of alpha-b. Because sorting receptors typically require the formation of multivalent interactions, this motif along with the alpha segments defined here could play a role in this aspect of PEX19 function. Neurospora genetics Neurospora strains were constructed according to standard methods. For the expression of PEX3 and PEX19 variants in Neurospora , genomic fragments encompassing these genes were introduced into the pBM60 vector and targeted to the his3 locus [58] in pex3 or pex19 mutant backgrounds. An HA-epitope tag was introduced into both genes. Mutants were constructed in these genomic fragments according to standard methods. The his3 -recipient strains also expresses mCherry-PTS1 from the csr1 locus [59] . Plasmids, Neurospora strains and primer sequences can be found in Supplementary Tables 1–3 , respectively. Protein expression and purification PEX19, GET3 and PEX3 lacking the N-terminal TMD (amino acids 39–623) were expressed from the pET15b (Novagen) vector in Escherichia coli BL21 (DE3, Stratagene) and purified on Ni-NTA resin as recommended by the manufacturer (Qiagen). For the production of biotinylated PEX3, an AviTag (GLNDIFEAQKIEWHE) was introduced into the N-terminus of PEX3 and the protein was co-expressed with the BirA biotin ligase (pBirAcm plasmid, Avidity). For biotinylation, Luria broth (LB) medium was supplemented with 50 μM biotin. Recombinant chaperones used in the cell-free reaction were either dialyzed against Buffer H (20 mM HEPES, pH 6.8, 50 mM KOAc, 200 mM sorbitol, 1 mM MgCl 2 ) or purified by size-exclusion chromatography using a Hi-load 16/60 Superdex 200 prep grade column (GE Healthcare) equilibrated in Buffer H. Cell-free chaperone assay GFP-TA fusions were constructed in the pT7 vector (Thermo Scientific), and mRNA was prepared from this template using the mMessage mMachine T7 Transcription Kit (Ambion). The mRNA was purified with MEGAclear columns (Ambion). Unless otherwise indicated, translation reactions were carried out using the 1-Step Human Coupled IVT Kit—DNA (Thermo Scientific) according to manufacturer’s instructions with the following modifications: for each reaction, 6.25 μl HeLa lysate, 1.25 μl accessory proteins, 2.5 μl reaction mix and 1 μl mRNA (300 ng μl −1 ) were combined with 5 μM of chaperone proteins or an equivalent volume of Buffer H to a final volume of 13.5 μl. Translation reactions were conducted for 2.5 h and western blotting was used to control for levels of protein expression. In Fig. 1c (bacterial translation) and Fig. 1i , translation was carried out with the PURExpress Bacterial In Vitro Protein Synthesis Kit (NEB). For gel filtration analysis, reactions were scaled up to 100 μl, centrifuged at 1.5k g for 2 min and the supernatant was analysed by fast protein liquid chromatography using a Superdex 200 10/300 GL column (GE Healthcare) equilibrated in Buffer H. Ten μg of BSA was added to 500 μl fractions from the gel filtration and the mixture was precipitated by addition of 125 μl of 6.1 N TCA. After incubation at 4 °C for 1 h, the mixture was centrifuged at 14k g for 20 min. The pellet was washed twice with 500 μl ice-cold acetone, dried at 95 °C, resuspended in 100 μl loading buffer and analysed by SDS–polyacrylamide gel electrophoresis (PAGE) and western blotting. Cell-free peroxisome targeting Peroxisomes were prepared from frozen mycelium of a Neurospora strain expressing mCherry-PTS1, as previously described [60] . Briefly, 500 μl of Buffer H containing protease inhibitor cocktail (Roche) and 1 mM PMSF (phenylmethylsulphonyl fluoride) was added to a volume of 250 μl of frozen mycelium powder. The mixture was thawed on ice for 15 min, passed through a 40-μm cell strainer (Falcon) and centrifuged at 0.4k g for 2 min to remove cell debris. Two hundred μl of the supernatant was centrifuged at 6k g for 2 min and the pellet was washed in 200 μl of Buffer H under the same conditions. The peroxisome-enriched pellet fraction was resuspended in 50 μl of Buffer H and 2.5 μl of these peroxisomes were added per translation reaction. Targeting reactions were carried out for 30 min at 30 °C. Mammalian cell microinjection mRNA for the indicated fusion proteins was prepared as described above and microinjected into natural rat kidney cells at a concentration of ~500 ng μl −1 . Microinjection was carried out using an Eppendorf FemtoJet microinjecter and a Leica micromanipulator. For experiments where ER was labelled, mRNA encoding mCherry-KDEL [61] was co-injected with the indicated GFP-TMD mRNA. Where peroxisomes are labelled, cells were pre-injected with recombinant mCherry-PTS1 at a concentration of 5 mg ml −1 and injected with the indicated mRNA ~18 h later. Mitochondria were labelled using MitoTracker Red FM according to manufacturer’s (Invitrogen) instructions. Carbonate and detergent extraction After cell-free TA protein targeting, two reaction equivalents were brought to a volume of 250 μl with Buffer H and peroxisomes were sedimented by centrifugation at 16k g for 10 min. The pellet was washed once with 300 μl Buffer H, resuspended in 90 μl of Buffer H and split into three identical samples. To these, we added 60 μl of Buffer H, 60 μl of 1 M sodium carbonate (final pH 11.0) or 60 μl of Buffer H with 1.5% (v/v) Triton X-100 (final concentration=1%). The reactions were incubated for 30 min at 4 °C and centrifuged at 100k g for 60 min to produce total (T), supernatant (S) and pellet (P) fractions, which were analysed by western blotting. Treatment with apyrase and ATPγS and GTPγS To deplete ATP, 50 U of apyrase (NEB) was added to reactions either before or after translation and the mixture was incubated for 5 min at 30 °C. ATPγS (Sigma) and GTPγS (Sigma) were added to reactions to a final concentration of 5 mM. The effect of these treatments on translation was assessed by anti-HA (Roche 12013819001) western blotting against model TA proteins, and the effect on standard targeting reactions was assessed by fluorescence microscopy as described below. Peroxisome immunoisolation and manipulation For immunoisolation ( Fig. 1i ), we used a strain expressing PMP22-HA and mCherry-PTS1. Peroxisomes were isolated from 500 μl of frozen powder as described above and added to sepharose beads (GE Healthcare) coated with anti-HA (Roche 11583816001). Binding was carried out for 60 min at 4 °C and beads were washed extensively with Buffer H. Western blotting was used to follow peroxisomes (anti-HA) and ER (anti-KAR2). For immunostaining ( Fig. 4c ), peroxisomes were isolated from 100 μl frozen powder as described above and resuspended in 100 μl of Buffer H-BSA (1 mg ml −1 BSA). Two μl of a biotinylated anti-HA antibody (Roche 12158167001) was added and peroxisomes were incubated for 60 min at 4 °C. Peroxisomes were washed twice and resuspended in 100 μl of Buffer H-BSA. Alexa-labelled streptavidin (Invitrogen S-11223) was added to the peroxisome suspension to a final concentration of 0.05 mg ml −1 and the mixture was incubated 60 min at 4 °C. Then, the peroxisomes were washed, resuspended in 50 μl Buffer H-BSA and examined by fluorescence microscopy. For treatment with protease, 1 μl (2 U) PreScission protease (GE Healthcare) was added to a 100 μl peroxisome suspension and the mixture was incubated for 90 min at room temperature. The sample was centrifuged at 16k g to produce pellet (P) and supernatant (S) fractions. The pellet fractions were further introduced into the cell-free targeting assay, or extracted with various chemical treatments as describe above. Flow cytometry Two cell-free reaction equivalents were diluted to a final volume of 200 μl with Buffer H and pelleted by spinning at 6k g . The pellets were resuspended with 250 μl Buffer H and analysed using flow cytometer (BD FACSAria Cell Sorter) and FLowJo software (Tree Star). To focus on organelles, the output was gated to exclude objects that produced significant forward and side scatter. Pull-down assay for PEX3/PEX19 interaction Biotin-PEX3 was purified from a crude E. coli lysate by direct binding to Streptavidin agarose beads (Novagen) for 60 min at 4 °C followed by extensive washing with Buffer H. The pull-down assay was conducted in Buffer H containing 1 mg ml −1 BSA. An approximately threefold molar excess of PEX19 was added to beads containing 4 μg of PEX3 (7.5 μl of packed bead volume) in a total volume of 45 μl. This mixture was incubated for 60 min at room temperature and washed three times with 500 μl Buffer H. Beads were pelleted and bound protein was analysed by SDS–PAGE and staining with Coommassie Brilliant Blue (Sigma). Interaction between PEX3 and cargo-loaded PEX19 Magnetic beads were prepared according to manufacturer’s instructions (Invitrogen, dynabeads M-270). Briefly, 6 mg of beads was suspended in a total volume of 600 μl with anti-HA antibodies (Roche 11867423001) at a final concentration of 50 μg ml −1 . After antibody coupling, the beads were washed and resuspended at a concentration of 10 mg ml −1 . For each pull down, one TMD-PEX26 translation reaction containing PEX19 variants (13.5 μl) was centrifuged at 0.2k g for 2 min to remove large debris. Approximately 5 μg of Biotin-PEX3 was added to the supernatant and Buffer H containing 1 mg ml −1 BSA was added to bring the volume to 65 μl. Thirty μl of prepared beads was added and this mixture was incubated for 30 min at room temperature. Beads were washed once with 400 μl Buffer H, once with 200 μl Buffer H containing 1% digitonin (Sigma), twice with 200 μl Buffer H and then once with 200 μl Last Washing Buffer (Invitrogen). Beads were boiled in SDS–PAGE loading buffer, after which TMD-PEX26 and PEX3 were analysed by SDS–PAGE and western blotting. Surface plasmon resonance All the proteins used for SPR analyses were purified by size-exclusion chromatography using a Superdex 200 10/300 GL column (GE Healthcare) equilibrated in HBS-EP buffer (10 mM HEPES, 150 mM NaCl, 3 mM EDTA, 0.05% Tween 20, pH 7.4). Biotin-PEX3 was immobilized onto a Streptavidin sensor chip (GE Healthcare), and the binding of alpha-mCherry proteins was monitored with a BIAcore 3000 instrument (GE Healthcare). Sensorgrams were recorded at 25 °C at a flow rate of 15 μl min −1 in HBS-EP buffer. PEX3 was regenerated using 0.05% SDS in HBS-EP. Quantitative western blotting Single HA-tagged PEX19 and TMD-PEX26 (ΔTMD; Supplementary Fig. 2 ) and triple HA-tagged PEX3 and TMD-PEX26 (ΔTMD; Supplementary Fig. 3a ) were expressed and purified from E. coli as described above. The indicated recombinant proteins were mixed at a 1:1 molar ratio and analysed by SDS–PAGE and staining with Coommassie Brilliant Blue. The same mixture was diluted 20-fold and analysed by SDS–PAGE and quantitative western blotting using the LI-COR Odyssey imaging system. For analysis of the ratio of TMD-PEX26 to PEX3 ( Supplementary Fig. 3b ), targeting reactions were extracted with sodium carbonate as described above and subjected to quantiative western blotting using the LI-COR Odyssey imaging system. Western blotting The following antibodies were used for enhanced chemiluminescence western blotting: to detect the HA epitope, horseradish peroxidase (HRP)-conjugated rat monoclonal anti-HA antibodies (Roche 12013819001, 1:2,000) were used. To detect mCherry, mouse monoclonal anti-mCherry antibodies (Clontech 632543, 1:1,000) followed by HRP-conjugated sheep anti-mouse IgG antibodies (GE Healthcare NA931-1ML, 1:10,000) were used. To detect KAR2, rabbit polyclonal anti-KAR2 antibodies (gift of Frank Nargang, 1:10,000) followed by HRP-conjugated goat anti-rabbit IgG antibodies (Jackson ImmunoResearch Laboratories 111-035-003, 1:20,000) were used. HRP-conjugated Streptavidin (Thermo Scientific 21130, 1:2,000) was used in enhanced chemiluminescence western blots against biotinylated proteins. For quantitative western blotting, anti-HA rat monoclonal antibodies against the HA epitope (Roche 11867423001, 1:2,000) followed by IRDye800CW goat anti-rat IgG antibodies (LI-COR 926-32219, 1:5,000) were used. Full-scan images of the western blots and gels used in the figures are shown in Supplementary Fig. 16 . Image acquisition and quantification The micrographs shown in Fig. 1b,f,h , Fig. 2a,b , Fig. 3f,h , Fig. 4b,c,f and Supplementary Fig. 6b,c were taken using an epifluorescence microscope (BX51; Olympus) equipped with a × 100/1.4 NA (numerical aperture) oil immersion objective (UplanSapo) and a digital camera (Coolsnap HQ; Photometrics) controlled by Metamorph software. Where GFP aggregates are shown, ImageJ ( http://rsb.info.nih.gov/ij/ ) was used to create a maximum projection of 10 images. For peroxisome targeting assay, 8–10 randomly chosen large peroxisomes were photographed for each experiment. Two representative images for peroxisome targeting assays are shown for each reaction condition. In experiments where targeting activities are compared, images were obtained using the same microscope and camera settings. The images shown in Fig. 1a,i , Fig. 2c and Supplementary Fig. 6a were acquired using a Leica SP5 inverted confocal microscope equipped with a × 100/1.4 NA objective. The images shown in Supplementary Fig. 10 were acquired using a Nikon Microlambda Spinning Disc confocal microscope equipped with a × 100/1.4 NA objective. Aggregates were quantified using the ‘Analyze Particle’ function in ImageJ. All the figures were created using Photoshop and Illustrator software (Adobe). How to cite this article: Chen, Y. et al. Hydrophobic handoff for direct delivery of peroxisome tail-anchored proteins. Nat. Commun. 5:5790 doi: 10.1038/ncomms6790 (2014).